PhyloPhlAn is a new method for improved phylogenetic and taxonomic placement of microbes New microbial genomes are constantly being sequenced, and it is crucial to accurately determine their taxonomic identities and evolutionary relationships. Here we report PhyloPhlAn, a new method to assign microbial phylogeny and putative taxonomy using >400 proteins optimized from among 3,737 genomes. This method measures the sequence diversity of all clades, classifies genomes from deep-branching candidate divisions through closely related subspecies and improves consistency between phylogenetic and taxonomic groupings. PhyloPhlAn improved taxonomic accuracy for existing and newly sequenced genomes, detecting 157 erroneous labels, correcting 46 and placing or refining 130 new genomes. We provide examples of accurate classifications from subspecies ( Sulfolobus spp.) to phyla, and of preliminary rooting of deep-branching candidate divisions, including consistent statistical support for Caldiserica (formerly candidate division OP5). PhyloPhlAn will thus be useful for both phylogenetic assessment and taxonomic quality control of newly sequenced genomes. The final phylogenies, conserved protein sequences and open-source implementation are available online. The reconstruction of evolutionary relationships (phylogeny) from DNA sequences is one of the oldest challenges in bioinformatics. Microbial phylogenies in particular are crucial for comparative genomics and understanding selective pressures in rapidly evolving single-celled organisms [1] ; microbial systematics also relies on the precise definition of a comprehensive microbial tree of life [2] . Whole-genome phylogenies are needed for taxonomic assignment of newly sequenced genomes, detection of horizontally transferred genes [3] and studying selection of genes, pathways [4] and pathogen mutations during disease outbreaks [5] . Accurate phylogenetic trees are also vital for estimating the microbial biodiversity of entire communities and relating it with environmental factors or human disease [6] . Although a wide range of methods have been described for aligning and reconstructing trees from individual peptide sequences, none to date have scaled to produce a highly resolved microbial phylogeny that takes full advantage of the millions of genes and thousands of genomes now sequenced. The microbial tree of life has long been of particular interest; gene- and protein sequence-based approaches at its reconstruction antedate modern genomics [7] . The 16S rRNA gene (subsequently abbreviated as 16S) is historically the most adopted phylogenetic marker [8] , but other single genes have been used for the same task [9] . Although differences can certainly arise between gene-focused and genome-focused phylogenies for any one marker, this has generally not precluded the biological utility and overall accuracy of bifurcating whole-genome trees [10] . While 16S databases, and thus phylogenies, include millions of sequences covering a substantial fraction of all microbes [11] , [12] , relying on any single gene lacks phylogenetic resolution at evolutionarily short time scales, preventing differentiation of closely related organisms [13] , and mutations or lateral transfers in any single gene may not be well correlated with organismal evolution [14] . As whole-sequenced genomes have become more abundant, the most successful recent approach for selecting markers for whole-genome phylogenetic reconstruction is based on the concatenated sequences of 31 manually curated conserved proteins [15] . This and other multi-gene methods have greatly improved the accuracy and resolution of the resulting microbial trees [16] when appropriate alignment and tree reconstruction methods are combined with the target sequences [17] , [18] . Proteins previously selected for this process are mainly ribosomal (23 out of 31), making the method dependent both on manual curation and on a single (albeit critical) cellular machinery. This is not necessarily an ideal proxy for organismal evolution, particularly given different rates of evolution among gene lineages [19] , [20] , [21] , [22] , [23] , and it is thus of course desirable to select several markers as molecular clocks of differing rates (that is, slow for resolving deep branches, rapid for placing recent divergences). Furthermore, the protein selection method was neither automated nor extended beyond the 191 genomes then available, and the implemented approaches, AMPHORA (ref. 16 ) and AMPHORA2 (ref. 24 ), have not been expanded to include more than 31 (in bacteria) or 104 (in archaea) proteins and ~1,000 complete genomes. In combination with the principle of statistical consistency [25] , [26] , this suggests that the quality of a reconstructed species tree likely correlates with the size of integrated sequence data, and small marker sets may thus not be representative of the threefold larger current catalogue of draft and final genomes. The converse problem, accurate placement of newly sequenced genomes within a reconstructed phylogeny, presents a comparable challenge. Surprisingly, although well-studied methods for tree insertion are available for the 16S phylogeny [27] and for arbitrary peptide sequences [28] , their accuracy for automated taxonomic assignment has been minimally studied. Classification approaches based on raw sequence similarity with a best-hit policy between new and labelled sequences typically neglect topology, and have not been assessed as a tool for recommending taxonomic labels for new genomes [29] . Moreover, genomes can themselves be occasionally taxonomically mislabelled or misplaced, leading to the propagation of errors if not properly considered. As manual curation is impractical for the thousands of microbial genomes now being regularly sequenced, novel computational tools for taxonomic characterization are needed, incorporating accurate, highly resolved and comprehensive phylogenies in order to guarantee reliable analyses. In this work, we propose and validate a novel method for accurate microbial phylogeny reconstruction, detection of potentially mislabelled genomes and taxonomy assignment using this phylogeny for newly sequenced genomes. The approach automatically and efficiently identifies hundreds of conserved proteins from the current catalogue of >3,700 finished and draft microbial genomes and uses them to build a complete high-resolution phylogeny. We develop several measures for quantitatively assessing the quality of the resulting phylogenies, all of which indicate that sampling peptides from hundreds of proteins results in increased accuracy relative to available methods. As the phylogeny is able to resolve both very closely related strains and deep-branching candidate divisions, newly sequenced genomes can be automatically integrated and, in many cases, assigned taxonomy with high confidence. We thus determined taxonomy for 130 previously unassigned genomes and have detected 157 sequenced microbes likely to be taxonomically misannotated, 46 with high-confidence corrections. The fully automated pipeline is freely available and scales to thousands of more sequenced genomes, thus remaining applicable to future genomic and metagenomic investigations. A high-resolution tree of life incorporating 400 markers We present an automated, high-throughput method for generating high-resolution microbial phylogenies by automatically detecting and combining ubiquitously conserved bacterial and archaeal proteins. Proteins are initially selected from among 2,780 bacterial and 107 archaeal genomes in IMG (version 3.4) [30] , and each are tested for conservation among over 10 million genes. We assess phylogenies built from up to the 500 proteins spanning the greatest diversity, as measured by a preliminary 16S-based phylogeny [11] . Phylogenetic trees are generated from subsequences of these proteins concatenating their most informative amino-acid positions, each aligned separately (using MUSCLE [31] ), and reconstructed into trees using FastTree [32] and RAxML [28] (see Methods). The most accurate resulting tree of life is built using >4,600 aligned amino-acid positions sampled from 400 proteins ( Fig. 1 ). This incorporates the original ~2,900 genomes, 848 more from IMG 3.5 and IMG-GEBA 3.5 (as of February 2012 (ref. 30 ), and two additional genomes from candidate division OP1 (ref. 33 ) and the Caldiserica phylum [34] . In addition to placing these genomes, taxonomic assignments are refined, flagged or newly provided for a total of 262 genomes. PhyloPhlAn, the implementation of these methods, is generalizable to any set of genomes. The process can quickly re-identify the most conserved proteins in a genome set, although this is not needed for phylogenetic placement or taxonomy assignment for newly sequenced genomes. 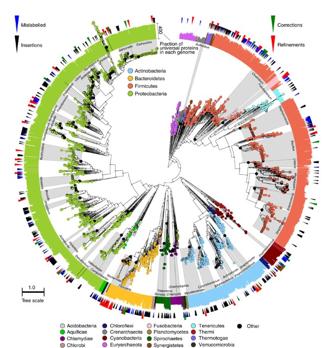Figure 1: A high-resolution microbial tree of life with taxonomic annotations. We reconstruct and validate a bacterial and archaeal phylogeny leveraging subsequences from 400 broadly conserved proteins determined using 2,887 genomes and applied on a total of 3,737 genomes. The tree is built using RAxML28, with organisms coloured based on phyla including at least five genomes. Scale indicates normalized fraction of total branch length. Grey labels indicate the lowest common ancestor of genera with at least 10 genomes (excluding predicted taxonomic mislabellings). External bar length represents the fraction of the 400 proteins contained in each genome. Red external triangles indicate genomes predicted by our method to be taxonomically mislabelled and confidently replaced; blue triangles indicate problematic labels that were refined but still did not fall within a fully consistent clade; green triangles indicate genomes whose incomplete taxonomic label we confidently refined; and black triangles indicate 566 genomes from IMG-GEBA that have been newly placed into the tree. Figure 1: A high-resolution microbial tree of life with taxonomic annotations. We reconstruct and validate a bacterial and archaeal phylogeny leveraging subsequences from 400 broadly conserved proteins determined using 2,887 genomes and applied on a total of 3,737 genomes. The tree is built using RAxML [28] , with organisms coloured based on phyla including at least five genomes. Scale indicates normalized fraction of total branch length. Grey labels indicate the lowest common ancestor of genera with at least 10 genomes (excluding predicted taxonomic mislabellings). External bar length represents the fraction of the 400 proteins contained in each genome. Red external triangles indicate genomes predicted by our method to be taxonomically mislabelled and confidently replaced; blue triangles indicate problematic labels that were refined but still did not fall within a fully consistent clade; green triangles indicate genomes whose incomplete taxonomic label we confidently refined; and black triangles indicate 566 genomes from IMG-GEBA that have been newly placed into the tree. Full size image The new phylogenies have high accuracy and consistency Unfortunately, no ground truth is available as a gold standard for assessing the topological accuracy of a phylogeny spanning billions of years of microbial evolution. As a surrogate, we quantitatively evaluate the consistency of our tree of life with respect to the IMG microbial taxonomy [30] . While no one taxonomy is perfect, this represents a well-accepted microbial categorization, as it has been extensively manually curated, and its genomic and phenotypic bases are well established [35] . Likewise, while we do not expect any phylogeny and taxonomy to match perfectly, they are unlikely to match by chance; thus, greater relative similarity is a reliable measure of increased accuracy. The first measure of phylogenetic quality we derive is the consistency or precision of a clade, which for the purposes of this manuscript is defined as a systematic group or leaves of a subtree sharing taxonomic labelling. Its precision is defined as the fraction of genomes within a subtree assigned to the same taxonomic group. For example, in our microbial tree of life ( Fig. 1 ), all Staphylococcus aureus genomes are contained in the same subtree without genomes from other organisms, thus achieving a precision of 1.0 (see Supplementary Methods equation (S1) ). Unsurprisingly, most well-studied model organisms achieve near perfect (>0.99) precision by our method, including Streptococcus pneumoniae , Salmonella enterica , Mycobacterium tuberculosis and Vibrio cholerae , among others. We next evaluate the recall of taxonomic clades based on the relative size of their largest taxonomically consistent subtrees (LTCS). The LTCS of a clade is defined as the phylogenetic subtree containing only members of that clade and spanning the greatest distance. That phylogenetic diversity represents the diameter of the LTCS (longest distance between leaves; see Supplementary Methods ), thus defining a clade’s recall as the fraction of its genomes within the LTCS diameter. Intuitively, a clade's recall quantifies how many of its genomes occur ‘close together’ within a phylogeny. All 20 phylum-level clades achieve perfect recall in our phylogeny, excluding Bacteroidetes at 0.99 due to an IMG 3.4 mislabelling discussed below. Thirty three of 36 (92%) class-level clades also have perfect recall, and 80 (82%) species-level clades possess recall >0.9. Notably, the Tenericutes phylum was rooted within the Firmicutes. The placement of the Tenericutes has been controversial since the inception of the tree of life, and several early trees indeed placed the ‘phylum’ within Firmicutes [36] , [37] . The recent concatenated proteins approach [16] also supports this inner rooting, and some reconstructions, such as RAxML ( Fig. 1 ) and the All-Species Living Tree project [38] , root the Fusobacteria within Firmicutes as well. The PhyloPhlAn placement of these well known yet challenging examples led us to examine the OP candidate divisions below and suggests that highly diverged clades are sometimes better classified by high-resolution protein sequence analysis than by phenotypic traits, let alone by the single 16S gene sequence. Choosing an optimal number of universal protein markers We next compare the accuracy of our approach with 16S and AMPHORA-based phylogenies across a wide range of parameters ( Fig. 2 and Supplementary Fig. S1 ). Specifically, we vary the number of conserved proteins considered from 5 to 500 ( Fig. 2a,b ) and the number of amino acids sampled from within these proteins from 30 to 4. Remarkably, we find that both phylogenetic precision and recall continue to increase at all taxonomic levels for reconstructions using up to 300 conserved proteins. Small improvements at higher phylogenetic levels continue as amino acids from up to 500 proteins are included, showing that it is indeed beneficial to employ as many conserved proteins as possible in the phylogenetic reconstruction procedure. This observation is most striking at the species level due to the fact that less universally conserved proteins provide conversely better resolution over short evolutionary time scales. PhyloPhlAn thus leverages this behaviour by combining many proteins with a core of highly conserved universal sequences, allowing both broad (phylum-level) and detailed (species-level) accuracy. 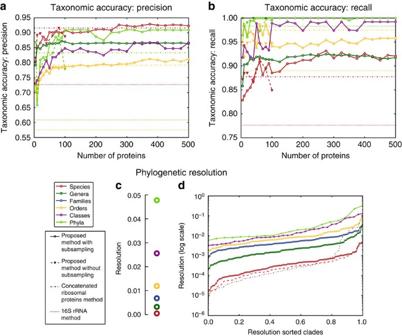Figure 2: Selecting informative subsequences improves the accuracy of phylogenetic tree reconstruction. As compared to a gold standard derived from the IMG taxonomy, both precision (a) and recall (b) of inferred phylogenies increase at all taxonomic levels as up to the 500 most conserved proteins are sampled (values averaged across all clades at each level). Comparison with full-length protein sequence phylogenies (up to 100 proteins) confirms that alignments sub-sampled at the most discriminative amino acids are both more accurate and more efficient. This approach outperforms single 16S rRNA gene phylogenies at all taxonomic levels, as well as trees based on curated ribosomal protein concatenation15,16for all but the most specific clades. (c) The relative phylogenetic diversity of all taxonomic levels is consistent across varying protein numbers and is on average remarkably logarithmic, providing quantitative support for the existing multi-level microbial taxonomy. (d) Relative phylogenetic diversity among individual clades at each taxonomic level, however, shows a tremendous range of diversities, with some underrepresented phyla comprising only as much sequence divergence among available genomes as some species. This suggests that while taxonomic levels are consistent on average, clade-specific diversity thresholds should be employed when linking phylogenetic divergence with individual taxonomic labels. Again, even the most diverse species reconstructed by this method are better resolved than those using the 16S rRNA gene alone, for which many demonstrate improbably high putative phylogenetic diversity. Figure 2: Selecting informative subsequences improves the accuracy of phylogenetic tree reconstruction. As compared to a gold standard derived from the IMG taxonomy, both precision ( a ) and recall ( b ) of inferred phylogenies increase at all taxonomic levels as up to the 500 most conserved proteins are sampled (values averaged across all clades at each level). Comparison with full-length protein sequence phylogenies (up to 100 proteins) confirms that alignments sub-sampled at the most discriminative amino acids are both more accurate and more efficient. This approach outperforms single 16S rRNA gene phylogenies at all taxonomic levels, as well as trees based on curated ribosomal protein concatenation [15] , [16] for all but the most specific clades. ( c ) The relative phylogenetic diversity of all taxonomic levels is consistent across varying protein numbers and is on average remarkably logarithmic, providing quantitative support for the existing multi-level microbial taxonomy. ( d ) Relative phylogenetic diversity among individual clades at each taxonomic level, however, shows a tremendous range of diversities, with some underrepresented phyla comprising only as much sequence divergence among available genomes as some species. This suggests that while taxonomic levels are consistent on average, clade-specific diversity thresholds should be employed when linking phylogenetic divergence with individual taxonomic labels. Again, even the most diverse species reconstructed by this method are better resolved than those using the 16S rRNA gene alone, for which many demonstrate improbably high putative phylogenetic diversity. Full size image Based on these results, we select the 400 most ubiquitous proteins to build our recommended tree of life, as gains in accuracy at any taxonomic level beyond this point were modest. For up to 100 proteins, the approach is also feasible using full-length protein sequences without any sub-sampling of alignment positions ( Fig. 2a,b ), but this provides no apparent benefit. It is also of note that the taxonomic levels achieving highest precision are the broadest (phyla) and the most specific (species), suggesting that those categories are both the most phylogenetically and taxonomically well defined. Difficulties in microbial taxonomic assignments at intermediate (class through genus) levels are well known and reflected by the substantial number of provisional clades among these levels (for example, 31 genomes in incertae sedis genera). We additionally compare our phylogenetic reconstructions with state-of-the-art methods based on the 16S gene and on 31 concatenated protein alignments [15] , [16] . While concatenating, ribosomal proteins greatly outperforms the 16S-based phylogeny as expected ( Fig. 2a,b ), both are outperformed at most phylogenetic levels by our methodology. The 31 ribosomal proteins [15] are remarkably precise and consistent at the species level, but performance decreases among all higher-level taxonomic clades. This may reflect the ambiguity of manual curation-based methods in assigning microbial taxonomy at intermediate levels, and emphasizes the need for automated approaches. Despite its ubiquity, the single 16S gene sequence proves highly noise prone as a sole marker for phylogeny ( Fig. 2a,b ). Specifically, on precision, our tree outperforms that of 16S-based approaches at every taxonomic level from species to phylum, averaging for clades with at least four genomes 92.5% for species, 86.6% for genera, 80.9% for families and orders, 86.8% for classes and 90.9% for phyla. Of 98 total species-level clades with at least four genomes, our final tree groups 80 (82%) of them with >0.9 precision, in contrast to only 58 (59%) in previous 16S gene-based approaches. We additionally assess that the reconstructed phylogeny is robust to horizontal gene transfer (HGT) by means of systematic gene transfer simulation ( Supplementary Fig. S2 and Supplementary Methods ). Even at extreme levels of synthetic HGT, this had a limited impact on inferred phylogenetic relationships as compared with the HGT-free PhyloPhlAn reference tree. Distances among leaf nodes in the HGT trees remained highly correlated with those in the original tree (correlation coefficients from 0.998 to 0.976 for 5 and 50% synthetic HGT, respectively). The strategy of including up to several hundred markers as diverse, repeated measures of divergence thus appears robust even to the high levels of HGT, although the magnitude of branch lengths in the reconstructed trees could be underestimated for clades with extensive HGT. Phylogenetic diversity at different taxonomic levels We next determine what the reconstructed phylogeny reveals about the diversity of taxonomic clades. We define a third quantitative measure, the relative phylogenetic diversity of a taxonomic clade within the phylogeny, as the total branch length spanned by the placement of all genomes within the clade. Averaging this overall for species, genera and so forth, determines the typical ‘diameter’ of each taxonomic level ( Fig. 2c ), which proves to be remarkably logarithmic. Classes typically capture half the sequence diversity of phyla (2.5% versus 4.8% of total diversity), orders half that of classes (1.2 versus 2.5%), and so forth. PhyloPhlAn again produces generally more discriminative phylogenies than existing methods, regardless of the number of proteins considered. The 16S gene alone, for example, places almost 15% of species in such a manner so as to include inconsistently high diversity. These behaviours represent averages, however, and are by no means consistent among clades ( Fig. 2d ). The most diverse taxonomic level, phyla, range from a maximum in Proteobacteria (one third of total diversity) to a minimum in Acidobacteria . At lower taxonomic levels, only a weak relationship between diversity and number of available genomes can be observed for families, genera and species ( Supplementary Fig. S3 , respective R 2 0.04, 0.22 and 0.30). Escherichia coli , for example, is the most sequenced species, but it is only the 18th most diverse. More surprisingly, genus- and species-level clades span more than two orders of magnitude in relative phylogenetic diversity: species with the highest diversity (>0.25%) included Buchnera , Prochlorococcus , Clostridium and Bacillus , whereas several Brucella species span very low relative phylogenetic diversity (<0.005%). All of these examples contain at least 12 sequenced genomes, and it is important to underscore that the true biological diversity of some clades may be underestimated if the genomes are insufficiently representative of the diversity within those clades. Analysing specific sub-clades of Bacteria and Archaea A recent study of 45 genomes in the Actinobacteria phylum [39] showed that a consistent and resolved phylogeny of this clade could not be achieved with rRNA genes (5S, 16S or 23S); one was inferred by combining several (155) concatenated genes together with features such as synteny and phylogenetic profiling. Our Actinobacteria reconstruction ( Fig. 3a ) achieves a fully consistent grouping of all 19 families, with the sole exception a Streptomyces genome phylogenetically included in Pseudonocardiaceae due to a known mislabelling [30] . Our method automatically flags this as a likely misannotation (red triangle in Fig. 3a ). All other genera and species included in the existing phylogeny [39] are correctly inferred here, confirming that this catalogue of 400 proteins allows accurate phylogenetic reconstruction without the need for additional genomic information. We then specifically investigate the Corynebacterium genus, as this clade has recently been phylogenetically characterized with conflicting topologies using the single 16S and rpoB genes [9] . In the PhyloPhlAn tree of the 31 Corynebacterium genomes ( Fig. 3b ), multiple strains in the same species always cluster together with relatively little divergence. Interestingly, intraspecies distances between complete and draft genomes are as small as those between complete genomes (see C. efficiens and C. aurimucosum ), confirming the PhyloPhlAn consistency in processing partially assembled genomes. 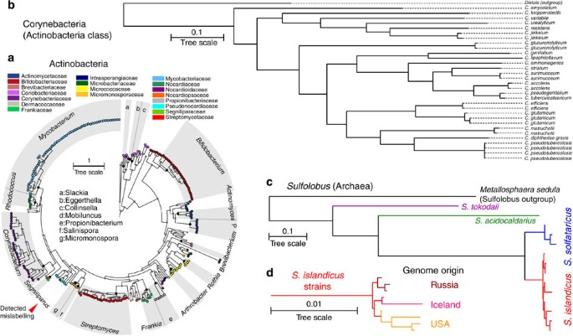Figure 3: Inferred phylum, genus and species phylogenetic trees. (a) The inferred Actinobacteria phylum subtree, with genomes coloured by family and genera annotated by root node. All 19 families are grouped consistently, which cannot be achieved by16Sgene sequences alone39. (b) TheCorynebacteriumgenus subtree, with highly concordant species and strain grouping not achieved by previous analyses9. (c) Archaeal genomes of genusSulfolobus, and (d) forS. islandicus, an inset of the inferred strain-level tree. For this particular organism, all nine genomes group consistently according to the geography of their site of origin. Figure 3: Inferred phylum, genus and species phylogenetic trees. ( a ) The inferred Actinobacteria phylum subtree, with genomes coloured by family and genera annotated by root node. All 19 families are grouped consistently, which cannot be achieved by 16S gene sequences alone [39] . ( b ) The Corynebacterium genus subtree, with highly concordant species and strain grouping not achieved by previous analyses [9] . ( c ) Archaeal genomes of genus Sulfolobus , and ( d ) for S. islandicus , an inset of the inferred strain-level tree. For this particular organism, all nine genomes group consistently according to the geography of their site of origin. Full size image The Archaea show similar accuracy ( Fig. 3c ); Sulfolobus is the genus with the greatest number of sequenced organisms (14), all representing thermoacidophiles isolated mainly from volcanic springs. Its phylogenetic tree is again monophyletic with respect to species and highlights interspecies diversity more than 20 × higher than intraclade diversity for S. solfataricus and S. islandicus . However, the low diversity in these two species does not affect the discriminative power of the subtree, as confirmed by the inset S. islandicus genomes ( Fig. 3d ). This strain-level phylogeny further exactly matches the distribution of these species, reflecting the geography of genomes sequenced from acid environments in American, Russian (7 genomes [40] ) and Icelandic (2 genomes) locations [41] . Phylogenetic placement of deep-branching organisms We next analyse the integration of two genomes from candidate divisions OP1 and Caldiserica (formerly OP5), which are particularly challenging cases lacking close relatives in the existing phylogeny, and the placement of similarly deep-branching representatives of divisions TM7 and OP11. Based on 16S data, OP1 was previously assessed as most closely related to Thermatoga ; TM7 was closest to Chloroflexi (specifically Chloroflexus auranticus [42] ), and OP11 was very deep branching [43] . A later study concatenated 44 highly conserved proteins and concluded that Coprothermobacter (family Thermodesulfobiaceae) was most closely related to the Dictyoglomi and Thermatoga, as well as confirming the Actinobacteria/Deinococcus-Thermus/Cyanobacteria/Chloroflexi grouping [44] . Our final phylogeny ( Fig. 1 and Supplementary Fig. S4 ) concurs with the confident subset of these previous placements and introduces a potentially deeper branching for Caldiserica. The description of the only current Caldiserica isolate, Caldisericum exile [34] , places it between the Proteobacteria and Acidobacteria phyla based on 16S data. Our results ( Supplementary Fig. S4 ) suggest a much deeper phylogeny, with Dictyoglomus and Thermotoga as sister phyla and consistent bootstrapping support (85%) for the combined Caldiserica- Coprothermobacter subclade; this placement should of course be explored by further targeted analyses. The placement of OP11 agrees with previous placements external to all major bacterial phyla [43] , but was based on a reduced core of 30 genes from a single draft genome of 417 proteins. Its placement is particularly challenging due to an unusually large fraction of short peptides (41.2% of proteins <100AA versus an average of 13.3% s.d. 5.7% for all genomes) and, as a result, the corresponding subtrees have low bootstrap support. Our phylogeny supports deep branching of Candidatus acetothermum autotrophum (OP1), in agreement with 16S and protein-based studies, but between Thermotoga and Archaea rather than Deinococcus–Thermus [33] , [43] . We group Actinobacteria, Deinococcus-Thermus, Cyanobacteria and Chloroflexi as sister phyla and propose that TM7, represented by only one genome, is not only closely related to Chloroflexi but possibly rooted within them, although the limited bootstrapping support (40%) suggests that this hypothesis needs independent validation. Efficiently expanding the tree of life with new genomes The identification of the 400 most conserved proteins in microbial genomes is made computationally tractable by our approach, but is still an expensive operation that is avoidable when creating or updating a phylogeny with new genomes. The PhyloPhlAn implementation stores a non-redundant database of the 400 proteins and their variants that is used for identifying them in new genomes by translated mapping with USEARCH [45] . Without any other prior information, a full tree of the 3,174 genomes in IMG version 3.5 is produced in under 2 h on a 16-CPU system using the FastTree application [32] . Even this step is typically unnecessary, however, as the pipeline also allows new genomes to be incorporated directly into an existing tree. IMG-GEBA 3.5 provides 566 new genomes without species labels, for example, and they have been integrated in this way and are indicated with black triangles in Fig. 1 . This most current phylogenetic tree is reconstructed with RAxML version 7.3.2 (ref. 28 ) in place of FastTree [32] to increase accuracy at the expense of computational time (620 instead of 2-CPU hours). Refining taxonomic assignments for new genomes As microbial genomes are now being sequenced by the hundreds, an important application of automated phylogenetic reconstruction is to suggest taxonomic labels for newly sequenced genomes. This is possible using guilt-by-association to transfer nearby taxonomic labels, and it is most straightforward when the genome is inserted within a monophyletic clade at any taxonomic level. Transfer is particularly confident when the genome’s distance from the lowest common ancestor of a monophyletic subtree is consistent with the subtree’s diameter (see Supplementary Methods ). Of the 566 IMG-GEBA genomes inserted above, when taxonomic information is stripped before PhyloPhlAn assignment, the pipeline assigns 56 to the species level, 164 at genus, 250 at family, 350 at order and 414 at class using the most stringent confidence threshold ( Supplementary Data 1 ). In many cases, newly sequenced genomes can be assigned at least partial taxonomy by a depositor, for example, to the family or genus level. This can be incorporated as additional information and either refined to a more specific level or flagged as suspect. Of the 566 partially labelled IMG-GEBA genomes, 51 are confidently refined to a species-level taxonomic assignment, whereas 20 of them are flagged as potentially misplaced and relabelled ( Supplementary Data 2 ). Thirty-six additional genomes are flagged as suspect without further confident refinement. These results are again obtained with the most stringent confidence threshold; results at more lenient thresholds are still informative but might require manual review. The accuracies of PhyloPhlAn’s three confidence levels are quantified on artificial data sets obtained by removing species-level labels from known genomes and re-imputing their taxonomy, with precision exceeding 80% for well-represented clades and 0 false positives at high confidence ( Fig. 4a ). 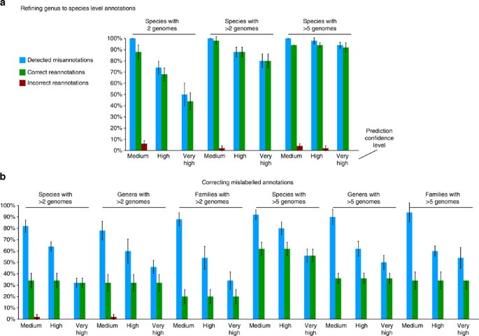Figure 4: Accuracy of correctly re-inferred taxonomic labels for artificially mislabelled organisms. Bar plots report the percentages (with s.d.) of successfully recovered cases. (a) For five iterations, 10 taxa are selected at random from species with two, more than two or more than five genomes, and their species-level label removed. The PhyloPhlAn phylogenetic tree (which is built without any taxonomic information) is then used to re-impute the removed labels at medium, high and very high-confidence thresholds. No incorrect refinements are produced at the highest confidence threshold, and average recall rates for species with at least three taxa exceed 90% at high confidence. (b) We repeat this procedure by mislabelling (rather than removing labels for) species, genus or family-level assignments. No false positives are produced at high or very high confidence, and only two at lower confidence (<1%). Figure 4: Accuracy of correctly re-inferred taxonomic labels for artificially mislabelled organisms. Bar plots report the percentages (with s.d.) of successfully recovered cases. ( a ) For five iterations, 10 taxa are selected at random from species with two, more than two or more than five genomes, and their species-level label removed. The PhyloPhlAn phylogenetic tree (which is built without any taxonomic information) is then used to re-impute the removed labels at medium, high and very high-confidence thresholds. No incorrect refinements are produced at the highest confidence threshold, and average recall rates for species with at least three taxa exceed 90% at high confidence. ( b ) We repeat this procedure by mislabelling (rather than removing labels for) species, genus or family-level assignments. No false positives are produced at high or very high confidence, and only two at lower confidence (<1%). Full size image Detection of taxonomic mislabelling and label assignment Our phylogenetic reconstruction method also suggests corrections to incomplete or misannotated entries in the current microbial taxonomy. Potential misclassifications are automatically flagged for inspection by checking whether a taxon is outside its largest consistent monophyletic subtree (see Methods); when possible, refinements are provided for genomes missing species-level labels by removing and re-imputing partial taxonomy. When applied to all 2,726 annotated genomes, potential corrections to the current microbial taxonomy range from simple typos to apparent phenotypic misclassifications. More than 5% (157) are detected as potentially misplaced, in addition to 410 genomes with incomplete taxonomy (totalling 17.8%). Twenty-six of the 157 flagged cases could be confidently reassigned to an equally specific taxonomic level, as well as a further 20 of the 114 genomes flagged during the IMG-GEBA insertions (58 more at less-strict confidence thresholds). Finally, between both genome sets, 71 of 445 genomes lacking detailed taxonomy are very confidently refined, resulting in the red (corrections), green (refinements) and blue (flags) annotations in Fig. 1 and the complete list of taxonomic corrections in Supplementary Data 3 . A striking example of misannotation in the existing taxonomy is the strain ATCC 43243 of Bacteroides pectinophilus , which we place well outside the otherwise fully consistent Bacteroidetes phylum. It instead falls within Clostridia, as verified by a manual phylogenetic analysis of the bacteroides [46] . This is fortunately the only phylum-level misclassification, with several of the others occurring at lower taxonomic levels associated with independent external confirmations. A representative subset of inferred taxonomic changes is reported in Table 1 . Table 1 Representative examples of taxonomic assignments inferred by PhyloPhlAn. Full size table We evaluate this approach by repeatedly artificially mislabelling 10 currently correct genomes and re-imputing them at increasingly strict confidence thresholds ( Fig. 4b ). This procedure is run five times each for randomly selected genomes in clades at increasing levels of specificity and with decreasing amounts of existing evidence (>5 to 2 supporting genomes). No false-positive imputations occur at the highest PhyloPhlAn confidence threshold among all 45 runs, and only 2 at medium confidence. Corresponding recall rates range from 78% and 82% in the most difficult cases to 94% in the best. We developed and validated an automated method for generating a highly resolved microbial tree of life that can be applied to taxonomically label newly sequenced microbial genomes. The method scales efficiently to incorporate all available finished and draft bacterial and archaeal genomes and leverages phylogenetic information from hundreds of proteins well conserved among microbial organisms. In the first comprehensive evaluation of the taxonomic precision and recall in microbial trees of life, the final phylogenetic trees produced by this method outperformed both the commonly employed single 16S gene [8] and state-of-the-art curated multiple protein approaches [15] , [16] . Total achievable accuracy continued to increase as informatively varying peptides were sampled from up to 500 total proteins, thus addressing potential pitfalls of single gene and manually curated methods and allowing the rapid taxonomic assignment of any newly sequenced microbial genome and the detection of 157 genomes likely to be currently misannotated. New microbial genomes are now being sequenced by the hundreds; thus, it is increasingly important to provide an accurate, high-resolution, automated framework for phylogenetic placement and recommended taxonomy. Long-standing phenotyping and biochemistry are vital for taxonomic validation, but it is impractical to perform these for all isolates in a high-throughput environment. PhyloPhlAn provides a systematic check for the thousands of genomes already sequenced and is compatible with draft genomes missing individual markers such as the 16S gene, microbes sequenced from uncultured samples [47] , partial assemblies from metagenomic data [48] and genomes with extensive HGT. Such genomes are often fragmentary, uncultured or phenotypically uncharacterized prior to sequencing and classification. Computational efficiency is also crucial for the increasing size of microbial genomics, and PhyloPhlAn scales at best (and typically) linearly and at worst quadratically with total genomes, making it suitable for much larger sequence compendia ( Supplementary Fig. S5 ). Finally, there are many theoretical motivations for improving large phylogenetic reconstructions by including many well-distributed genomes [49] , [50] , and PhyloPhlAn thus represents a means to efficiently employ the increasing catalogue of microbial genomes. Variations on this method have already been useful for efficient and high-throughput taxonomic assessment of whole uncultured communities [51] and can be crucial for mining meta'omic data sets [52] . Opportunities exist to further refine all of PhyloPhlAn's three primary steps: identifying informative conserved residues, reconstructing a species tree and inferring new genomes' putative taxonomy. We currently favour conserved proteins by drawing proportionally more residues from them, tending to identify residues that are ‘slightly saturated’ [53] . The parameters or method used to select these residues and the number of loci included could be optimized using holdout sequences or new genomes. Different tree reconstruction algorithms can be used with the selected residues, and this raises the possibility of evaluating additional evolutional models and tree-combining [54] or alignment-free [55] reconstructions. Likewise, different genome placement classifiers could be used to assign putative taxonomy. This is particularly of interst, as more advanced ortholog/paralog detetion methods and annotation-free identification of conserved target sequences may further improve accuracy on partial genomes derived from metagenomes or single-cell sequencing ( Supplementary Tables S1 and S2 ). The tasks enabled by a microbial tree of life with phylum-to-species accuracy include additional evolutionary and comparative genomic applications not covered in our initial analyses. For example, some microbial clades have very broad pan-genomes (for example, Prochlorococcus marinus with a pan-genome 4 × larger than its median genome), for which we could detect enrichments for specific genes, pathways or functionality within phylogenetically well-defined subtrees. When considering the entire tree of life, the relationship between functional and evolutionary distances can be compared for investigating convergent functional specialization of unrelated bacteria [56] or, conversely, divergence in recent speciation [57] . Overall, the high consistency achieved by this phylogenetic tree built using hundreds of well-conserved proteins provides a solid foundation for future high-throughput studies of taxonomy, comparative genomics, systematics and taxonomic classification relying on an accurate and comprehensive microbial tree of life. PhyloPhlAn reconstruction pipeline and availability The developed open-source software, documentation, tutorial, resulting data and supplemental information are available online and for download (PhyloPhlAn website [58] , with a copy in Supplementary Software). PhyloPhlAn implements all phylogenetic reconstruction steps (conserved protein detection, tree building and integration of new genomes into the tree, all described in the Supplementary Methods ) and taxonomic curation strategies (mislabelling detection, label imputation/refinement for new genomes and label imputation/refinement for detected mislabelling, described below). The PhyloPhlAn approach is based on the 400 most universal proteins that have been identified by off-line preprocessing of all available microbial genomes. The pre-processing steps include core gene identification [13] and merging core genes into universal protein families (described below), and ranking each protein family for ubiquitous conservation and covered diversity in the microbial domain ( Supplementary Methods ). Genomic input data All 2,887 sequenced microbial genomes were retrieved from the Integrated Microbial Genomes [30] (IMG) version 3.4 with corresponding coding sequence (CDS) calls, translated protein sequences and taxonomic assignments. Genomes were screened for length >50,000 nt, at least 50 CDSs, and at least 75% of the genome CDs. Fifty-one of the remaining genomes lacked a taxonomic label below the family level and were considered to be taxonomically uncharacterized. One-thousand two-hundred twenty-one 16S gene sequences representing IMG species were retrieved from Greengenes [11] . CDS to COG assignments and 16S rRNA gene annotations were downloaded from IMG and used only for identifying the 31 ribosomal proteins for re-performing the corresponding method [15] , [16] with these genomes as described in the Supplementary Methods (‘Building phylogenetic trees using 16S and ribosomal proteins’). The PhyloPhlAn pipeline was further tested on the 3,171 genomes from IMG 3.5 as of February 2012; 566 additional genomes not contained in IMG 3.5 were downloaded from IMG-GEBA [30] as of March 2012 and the genomes of candidate division OP1 [33] and Caldiserica [34] were retrieved from the GOLD database [59] (GOLD ids Gc02183 and Gi17125, respectively). Identification of core genes Our unsupervised pipeline identifies the most ubiquitous proteins in thousands of genomes while avoiding computationally infeasible brute-force pairwise sequence comparisons between all >10M microbial CDSs. The three main steps of the method are (i) identifying nucleotide-level core genes, that is, those consistently present in at least one low-diversity clade (approximately from species to family levels), (ii) finding strong amino-acid homologues between core genes to detect universal proteins conserved in multiple lineages and (iii) ranking these universal proteins based on the number of genomes containing them and the total diversity they span. For identifying core genes, we employed and expanded a previous method for hierarchically identifying CDS homologues by means of recursive clustering on a guide tree [13] , [51] . Each genome was first transformed into a collection of clustered CDSs. From each cluster, a single representative (seed) was selected. Seeds from all strain-level genomes in each species were compared using UCLUST [31] at 75% nucleotide identity to identify species-level core genes. We introduced several refinements to this step to make the identification procedure robust to missing genomic regions and errors in CDS calls and taxonomic assignment. To capture missing or unannotated CDSs, each seed was aligned by BLASTN against every raw genome, and high-confidence matches were added to the corresponding gene family clusters. To address draft genomes and misannotated open reading frames, we generalized the definition of core gene using a probabilistic model. The presence/absence of a gene family across a group of genomes was modelled as a beta function of expected posterior probability density. We selected gene families with a >95% probability of being core in each clade given a 5% missing gene rate from annotation and assembly errors (measured from missing 16S annotations), and propagated them to the next level of identification. Genomes assigned by IMG directly to the genus (or higher) level were not considered during species-level core identification, but were included subsequently. Once species core genes were determined, clustering and comparing gene families were recursively applied to successively higher taxonomic levels (from genus to phylum). Merging core genes into universal protein families To detect proteins with homologues in a large fraction of genomes, we performed a translated nucleotide search against the microbial proteomes for a reduced set of conserved core genes. Specifically, we selected the 50 most conserved core genes in each lineage at the highest level of the taxonomic guide tree covering a maximum of genomes, resulting in a catalogue of 39,000 CDSs. NCBI Blastx [60] (e-value <1e−50) generated a bipartite graph between core genes and amino-acid sequences. The proteomes of the 51 organisms without clear taxonomy (excluded from core gene identification above) were included in this translated search to permit downstream phylogenetic profiling. Unsurprisingly, several very similar sets of proteins were targeted by more than one core gene, when several amino-acid sequences were conserved in multiple lineages but were missing or substituted by functionally related proteins in specific clades. We thus binned together each set of proteins targeted by approximately the same set of core genes, initially evaluating three different approaches: intersection of the overlapping sets of target proteins, union or selection of the largest of those sets, in all cases thresholded at a minimum overlap of 95%, and maximum disjoint fraction at 5%. Preliminary evaluation showed that the final maximum cardinality approach was the most accurate, and we thus selected it for downstream analyses. The resulting fully disjoint catalogue of protein families comprised 513 sets of proteins, each present in at least 1,000 genomes. It is worth mentioning that the use of core genes rather than all gene calls for alignment against proteomes does not cause the misdetection of any ubiquitous proteins; any protein present in at least 1,000 genomes must be core in at least one genus level or higher clade, and the process takes possibly missing or misannotated CDSs into account [13] . Universal proteins are then ranked for ubiquitous conservation as described in the Supplementary Methods . Detecting potentially misannotated genomes Genomes that are phylogenetically rooted well outside the largest monophyletic subtree (that is, the LTCS) of their putative taxonomic clades are flagged as potentially mislabelled. This test is performed on all genomes within any clades (at any taxonomic level) containing at least four representative genomes; a reliable LTCS cannot be defined when fewer sequences are available. LTCS calculation and all subsequent taxonomic label comparisons are performed using only genomes for which a fully defined curated taxonomy is available. Let D be the ratio between the genome's distance from the LTCS and the 75th percentile of all within-clade distances. If D<1.0, the genome is not flagged. Similarly, let R′ be the ratio of two additional distances from the genome of interest, first to the closest genome in the LCA sharing the target level's taxonomic label, and second to the closest of any genome in the LTCS. R′ <1.0 indicates at least one other genome outside the LTCS supports the current label, in which case the genome is again not flagged. Genomes meeting neither of these criteria are flagged as potential misannotations at one of three different confidence levels. Let R′ be the fraction of the clade of interest included in the LTCS; high values of R′ reflect sub-clades that are consistent except for the genome under consideration. Genomes with D ≥2.0, R ′≥2 and R ′≥0.8 are flagged with very high confidence; genomes with 1.25< D <2.0, 1.5< R ′<2 and 0.7< R ′<0.8 receive high confidence; and flagged genomes not meeting these thresholds are annotated as medium-confidence misannotations. Medium-confidence assignments are thus still unlikely to be correct due to the lack of strong phylogenetic evidence supporting a putative taxonomic label. Inferring taxonomy for unlabelled or misannotated genomes Genomes with incomplete or absent manually assigned taxonomy, or whose taxonomic label has been flagged as inconsistent (as described above), can be provided with a putative improved label based on evidence from the surrounding phylogeny. By default, the pipeline will taxonomically re-profile only very high-confidence predictions. First, we identify the largest otherwise fully monophyletic subtree containing the genome of interest. If such a subtree exists (that is, if it consists of more than one taxon in addition to the target), the taxonomic label of this subtree is initially assigned to the genome with medium confidence. This confidence score is increased if the distance of the target genome from the other genomes inside the subtree is consistent with the overall distribution of intraclade distances. Specifically, the distance between the target and the closest other within-clade genome is compared to the distribution of all minimum pairwise distances between leaves in the subtree. If the target rank is within the 95th percentile, the relabelling is increased to very high confidence, and high confidence is assigned at the 90th percentile. If no such monophyletic subtree exists for a flagged or unannotated target, we reassign taxonomy only if the genome under investigation is extremely close to a well-defined genome. In particular, very high confidence is assigned for cases in which the distance of the closest fully characterized taxon is below the median of all closest pairwise distances in the same clade for the taxonomic level of interest or smaller than 0.001% of the total diversity in the tree. High confidence is assigned if the distance ranks between the 50th and 75th percentile, and medium confidence between the 75th and 90th percentiles. Genomes falling above the 90th percentile remain flagged, but no new putative taxonomy is automatically provided. How to cite this article: Segata, N. et al . PhyloPhlAn is a new method for improved phylogenetic and taxonomic placement of microbes. Nat. Commun. 4:2304 doi: 10.1038/ncomms3304 (2013).